The molecular structure of the left-handed supra-molecular helix of eukaryotic polyribosomes During protein synthesis, several ribosomes bind to a single messenger RNA (mRNA) forming large macromolecular assemblies called polyribosomes. Here we report the detailed molecular structure of a 100 MDa eukaryotic poly-ribosome complex derived from cryo electron tomography, sub-tomogram averaging and pseudo-atomic modelling by crystal structure fitting. The structure allowed the visualization of the three functional parts of the polysome assembly, the central core region that forms a rather compact left-handed supra-molecular helix, and the more open regions that harbour the initiation and termination sites at either ends. The helical region forms a continuous mRNA channel where the mRNA strand bridges neighbouring exit and entry sites of the ribosomes and prevents mRNA looping between ribosomes. This structure provides unprecedented insights into protein- and RNA-mediated inter-ribosome contacts that involve conserved sites through 40S subunits and long protruding RNA expansion segments, suggesting a role in stabilizing the overall polyribosomal assembly. In eukaryotes up to a quarter of the cellular mass comprises ribosomes which perform protein synthesis, a process during which many ribosomes may bind simultaneously to a messenger RNA (mRNA) molecule [1] and thus form polysomes. These were first visualized in the mid 1960s (ref. 2 ) and often form double-row and helical arrangements [3] , [4] , [5] , [6] , [7] . First three-dimensional (3D) insights into prokaryotic and eukaryotic polysomes have been gained recently at moderate resolution [8] , [9] but a detailed analysis of their 3D organization was not possible yet with respect to the precise inter-molecular interactions between the ribosomes. Moreover the mRNA conformation within these supra-molecular structures has remained unclear, while it is well-known for individual ribosome particles from various crystal structures of pro- and eukaryotic ribosomes. The present study focuses on the analysis of the helical organization of higher-order poly-ribosome assemblies, while previous work [9] analyzed the more general organization of polysomes in various open, spiral, linear or planar structures of small- to medium-sized ribosome clusters. By using a combination of high-resolution cryo electron tomography (cryo-ET), sub-tomogram averaging of the polysomal ribosome s and molecular modelling using available crystal structures we derive the full pseudo-atomic structure of a helical higher-order eukaryotic polyribosome. This structure allows the detailed description of a representative complex, which comprises 23 ribosomes and has a molecular weight of about 100 MDa, one of the largest asymmetric structures of a poly-complex ever determined to high resolution. The improved resolution over previous work and the detailed atomic modelling allows an in-depth analysis at the molecular and atomic level of poly-ribosome assemblies, which was not possible before (also because high-resolution structures of eukaryotic ribosomes were not available at the time), thus strongly extending the level of interpretation as compared with earlier data [9] , and providing new mechanistic insights with important functional implications. The structure presented here provides unprecedented insights into protein- and RNA-mediated inter-ribosome contacts and by inferring the topology and conformation of the mRNA within the polysome assembly. In particular, the structure provides a first precise description of the helical parameters, which we show are related with the helical properties of the mRNA strand and the formation of a continuous mRNA channel, a new concept which was never described before. Second, the precise description of the inter-ribosomal contacts turns out to be the key for understanding poly-ribosome assembly, which allows protein synthesis to occur from parallelized machineries. These translation machineries are visualized here in an integrated manner across resolutions and scales from the cellular assembly level down to the atomic level, and across functional states of initiation, elongation and termination steps. 3D reconstruction of the eukaryotic polysome Eukaryotic polysomes were obtained using a continuous cell-free wheat germ translation system (CECF) [10] and analyzed in the frozen-hydrated state by cryo-ET ( Supplementary Fig. 1 ), using a CCD camera or a high-sensitivity direct electron detector (Complementary Metal-Oxide Semiconductor (CMOS)), which provided significantly improved image contrast [11] , [12] and helped pushing the resolution of the final reconstructions (see Supplementary Fig. 2 for a comparison of classical CCD data and new CMOS data, illustrating the advance gained in resolution; see methods for detailed data collection parameters and software used, and for image processing procedures). To summarize, five technical aspects can be highlighted here, which helped obtaining well-defined tomograms: (i) usage of a CMOS camera providing improved contrast at any voltage (including at 150 kV) with low total dose (30 e − Å −2 ), (ii) template-free maximum-likelihood-based sub-tomogram averaging from individual particles, (iii) no sub-tomogram merging between different tomograms to keep best data consistency (especially with regard to the defocus as no contrast-transfer function correction was done; that is, instead of several thousands only 106 particles for the polysome shown in Fig. 1 , which gave a well-resolved map considering the relatively small amount of particles), (iv) dual-tilt series with reduced missing wedge effects used for validation of the 3D alignment parameters during sub-tomogram averaging and fitting, and (v) over-sampling (3.4 Å per pixel) for final refinements and 3D reconstructions (see raw tomogram in Supplementary Fig. 2 before sub-tomogram averaging). The sub-tomogram averaging of the individual polysomal ribosomes provided a well-defined map, which was placed back into each ribosome position within the tomogram ( Fig. 1a ). This structure was interpreted at the atomic level by fitting the available crystal and cryo electron microscopy (cryo-EM) structures of eukaryotic ribosomes [13] , [14] ( Fig. 1b ), which gives a full pseudo-atomic model of this molecular assembly. 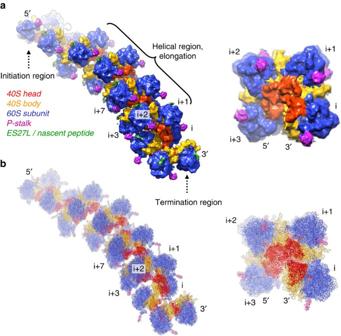Figure 1: Molecular structure of the left-handed supra-molecular helix formed by eukaryotic polyribosomes. (a) 3D reconstruction of eukaryotic polysomes obtained from cryo electron tomography and sub-tomogram averaging, revealing a left-handed supra-molecular organization. Colour code: 60S subunit, blue; 40S head, red; 40S body, yellow; P-stalk, pink; expansion segment ES27L and nascent peptide, green. The ribosome-loading region at the 5′ end of the mRNA is indicated, as well as the 3′-end region where translation terminates. The central part of elongating ribosomes forms a tightly packed helical array, as seen also from the 3′-end view on the helical axis of the polysome (right panel). The upstream ribosomes on the mRNA are indicated (i+1 and so on) with respect to the leading ribosome (i). (b) Atomic model of the 100 MDa polysome complex derived from fitting the available crystal and cryo-EM structures of eukaryotic ribosomes13,14,31, 5′ and 3′ ends are annotated; 3′-end view (right panel) as ina, showing that four ribosomes per turn form the left-handed helix. Figure 1: Molecular structure of the left-handed supra-molecular helix formed by eukaryotic polyribosomes. ( a ) 3D reconstruction of eukaryotic polysomes obtained from cryo electron tomography and sub-tomogram averaging, revealing a left-handed supra-molecular organization. Colour code: 60S subunit, blue; 40S head, red; 40S body, yellow; P-stalk, pink; expansion segment ES27L and nascent peptide, green. The ribosome-loading region at the 5′ end of the mRNA is indicated, as well as the 3′-end region where translation terminates. The central part of elongating ribosomes forms a tightly packed helical array, as seen also from the 3′-end view on the helical axis of the polysome (right panel). The upstream ribosomes on the mRNA are indicated (i+1 and so on) with respect to the leading ribosome (i). ( b ) Atomic model of the 100 MDa polysome complex derived from fitting the available crystal and cryo-EM structures of eukaryotic ribosomes [13] , [14] , [31] , 5′ and 3′ ends are annotated; 3′-end view (right panel) as in a , showing that four ribosomes per turn form the left-handed helix. Full size image Structure of the left-handed supra-molecular polysome helix The structure of the higher-order polysomes shows that they form left-handed supra-molecular helices ( Fig. 1 ), similar to some helical polysomes from human cells [9] , but the present high-resolution tomogram reconstruction now allows defining the precise helical parameters. The polysome structure forms a single-start left-handed supra-molecular helix with idealized parameters of ~570–580 Å diameter, ~four ribosomes per turn, a helix pitch of 330 Å and an axial rise of ~83 Å. Because the mRNA progresses in a defined direction it generates a polarity within the helix, which corresponds to the 5′ and 3′ ends of the open reading frame: these are located at each end of the supra-molecular helix ( Fig. 1 ). The helical array organization of the large central region of polysomes is based on closely positioned ribosomes, but we observe that the polysome structure deviates from the ideal helix at either ends. This leads to partially open helical segments in which the ribosomes pack less tightly and in a more open and irregular way; functionally, this corresponds to the loading region with the newly incoming ribosomes at the 5′ side of the mRNA in the initiation region and the termination region at the 3′ end ( Fig. 1a ). Characteristic contact sites between consecutive ribosomes Within the core region of the polysome, the ribosomes contact each other always through the 40S subunits which are oriented inwards ( Fig. 1 ), and through parts of the 60S subunits, revealing a significant shape complementarity between ribosomes when packed as a helical array. A detailed analysis of the interactions between neighbouring particles reveals three major contact sites ( Fig. 2 ), two of which involve adjacent 40S subunits and are common to most ribosomes, while the third is observed more rarely (see below). The total interaction surface area between adjacent ribosomes is in the range of ~98,000 Å 2 ; a total of ~196,000 Å 2 of each ribosome is involved in interactions, which sums up to ~30% of the total ribosome surface ( Fig. 2a ). The particularly large inter-ribosome surface areas explain the stability of polysome assemblies, which are seen in cellular structures and which withstand sucrose gradients generally used for purification and characterization. 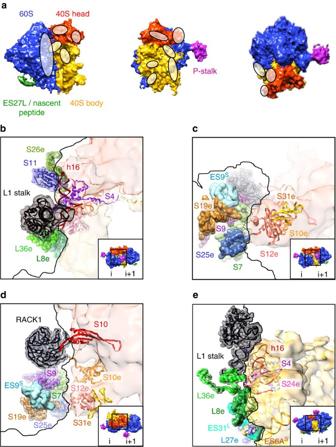Figure 2: Characteristic interaction sites between adjacent ribosomes in the polysome complex. (a) Inter-ribosome contact regions displayed on the back, 40S-solvent and top views of the individual ribosomes (the sub-tomogram averaged map is colour coded as inFig. 1). (b–e)Schematic views into the atomic model of the polysome complex at the inter-ribosome contact regions; the inserts indicate the region and viewing angle of the contact site within the polysome (more detailed figures are provided asSupplementary Fig. 3; see also the list of main contacts inTable 1). The sub-tomogram map in light colour delineates the individual ribosome on the right for which ribosomal proteins are shown in backbone representation, while proteins and rRNAs of the left ribosome are given as van der Waals surface representations to better distinguish the key elements of the two ribosomes participating in the interfaces. (b) The first contact site involves helix h16 of the 18S rRNA of the (i+1) ribosome and the L1-stalk region of (i) ribosome (ribosomal proteins involved in interactions are coloured, the remainder of the ribosome is in grey). (c,d) The second typical interaction region comprises head-to-head interactions between adjacent 40S subunits and involves the RACK1 protein and several other ribosomal proteins as annotated. (e) The extended contact site corresponds to contacts between neighbouring 60S and 40S ribosomal subunits that form on the concave side of slightly bent helical polysomes. In addition to the ribosomal proteins indicated, this also involves expansion segments ES31L, ES6ASand ES6BS. Figure 2: Characteristic interaction sites between adjacent ribosomes in the polysome complex. ( a ) Inter-ribosome contact regions displayed on the back, 40S-solvent and top views of the individual ribosomes (the sub-tomogram averaged map is colour coded as in Fig. 1 ). ( b – e) Schematic views into the atomic model of the polysome complex at the inter-ribosome contact regions; the inserts indicate the region and viewing angle of the contact site within the polysome (more detailed figures are provided as Supplementary Fig. 3 ; see also the list of main contacts in Table 1 ). The sub-tomogram map in light colour delineates the individual ribosome on the right for which ribosomal proteins are shown in backbone representation, while proteins and rRNAs of the left ribosome are given as van der Waals surface representations to better distinguish the key elements of the two ribosomes participating in the interfaces. ( b ) The first contact site involves helix h16 of the 18S rRNA of the (i+1) ribosome and the L1-stalk region of (i) ribosome (ribosomal proteins involved in interactions are coloured, the remainder of the ribosome is in grey). ( c , d ) The second typical interaction region comprises head-to-head interactions between adjacent 40S subunits and involves the RACK1 protein and several other ribosomal proteins as annotated. ( e ) The extended contact site corresponds to contacts between neighbouring 60S and 40S ribosomal subunits that form on the concave side of slightly bent helical polysomes. In addition to the ribosomal proteins indicated, this also involves expansion segments ES31 L , ES6A S and ES6B S . Full size image Figure 2 shows the three main inter-ribosome contact sites in a simplified way (a full description is provided in Supplementary Fig. 3 and a list of the main ribosomal proteins and ribosomal RNAs (rRNAs) involved is provided in the Table 1 ). The core of the first contact site is formed by helix h16 (18S rRNA) from the 40S subunit of the (i+1) ribosome and the L1-stalk of the (i) neighbour ribosome ( Fig. 2b ; ribosome number annotations are indicated in Fig. 1 ). In addition, protein S28e (40S of the (i) ribosome) interacts with the tip of helix h16 ( Supplementary Fig. 3 ), and the L1-stalk of the 60S subunit interacts with protein S4 and the central part of helix h16 of the (i+1) 40S subunit (the ribosomal protein annotation follows the Yusupov nomenclature [13] ). These contacts are extended by proteins S1e, S11 and S26e interacting with the tip of h16 and S4 ( Supplementary Fig. 3A ). Thus, helix h16 forms contacts with two regions of the neighbor ribosome that are next to the E-site transfer RNA and the 40S platform from where the mRNA emerges during the translocation process. Table 1 Main contacts between ribosomes in helical polysomes. Full size table The second typical contact site comprises head-to-head interactions between adjacent 40S subunits ( Fig. 2c,d ). One contact region comprises the exposed protein S10e (and S12e) on the 40S head, which interacts with proteins S7 and S19e (extended by S9 and S25e on the 40S platform region, Supplementary Fig. 3B ) and expansion segment (ES) ES9 S ( Fig. 2c ). A second contact involves protein receptor for activated C-kinase 1 (RACK1) which is in vicinity of protein S10 of the (i+1) ribosome 40S head ( Fig. 2d ). Functionally, this contact site appears important because RACK1 interacts with the polysome-associated protein Scp160, which promotes mRNA binding [15] , [16] . RACK1 is involved in the PKC (protein kinase C) dependent phosphorylation of initiation factor 4E, which promotes polysome-dependent de novo protein synthesis [17] . It is clear that within the polysomal complex, RACK1 is in part hidden by the neighbour protein S10, thus possibly preventing PKC and other proteins from binding ( Fig. 2d ). An additional third interaction region ( Fig. 2e ) can be observed on the concave side of the slightly bent region of the helical polysome where contacts of sites 1 and 2 are extended and reinforced by additional multiple interactions between neighbouring 60S and 40S subunits ( Supplementary Fig. 3C ; proteins L8e, L36e and the L1-stalk interact with proteins S4, S24e, L24e and the central region of h16). Protein L24e mediates an unexpected direct 60S–60S interaction through its long N-terminal α-helix that crosses the 40S subunit ( Supplementary Fig. 3C ). This contact region is further extended by ES elements, notably ES31 L which interacts with ES6A S , and ES6B S (18S rRNA) which contacts protein L8e. Role of rRNA ES in inter-ribosomal contacts The contacts mediated by rRNA ES elements represent a characteristic feature of the polysome structure. ES elements contain particularly long RNA structures protruding from the ribosome core and for which the function is essentially unknown. The inter-ribosome contacts observed here suggest that the ES elements contribute to stabilizing the overall polysome architecture. This is the case for the ES31 L —ES6A S interaction mentioned above. Another striking example is ES27 L . A density corresponding to the beginning of the RNA helix suggests that this prominent structural element is oriented towards the P-stalk region (protein P2 of the P0/P1/P2 complex) of the ribosome located one turn upstream of the helix. The P-stalk is actually well-defined in the sub-tomogram map, revealing that it is in proximity with the nascent peptide protruding from the ribosome one turn downstream (for example, P-stalk of (i+7) and ES27 L /peptide of (i+3) ribosomes in Fig. 1a ). Formation of a continuous mRNA channel The structure of the polysome complex allows inferring the path of the mRNA by connecting adjacent mRNA exit and entry sites on the 40S ribosomal subunits ( Fig. 3 ). Interestingly, rRNA helix h16 appears to serve as a walkway to guide the mRNA (not resolved here because of its single-stranded structure) from the mRNA exit site on the 40S subunit near the L1 region to enter the next following (i+1) ribosome ( Fig. 3a ). This suggests that the mRNA strand can directly connect the leading and the subsequent ribosomes. Because the mRNA exit and entry sites on the 40S ribosomal subunits are located close to the helical axis ( Figs 1a and 3a ), the mRNA path also adopts the same helical configuration as the supra-molecular helix formed by the ribosomes ( Fig. 3b ). This results in an overall continuous twist and curvature of the mRNA strand throughout the polysome. The reason for that is that the channel curvature is present in each individual ribosome and generates ¼ of a helical turn of the polysome. The local mRNA curvature in the mRNA channel of a ribosome then extends to the entire polysome. The supra-molecular arrangement thus builds up an almost continuous helical mRNA channel within the polysome. Consideration of mRNA base-pair length and inter-ribosome distances show that the measured average mRNA length is about 105 Å between consecutive ribosomes, consistent with the observation that up to 28 ribosomes are bound on the mRNA used here (975 nucleotide coding region, gives ~32–39 nucleotides per ribosome of which about half are inside the mRNA channel). This estimation is in agreement with the observation of tightly packed ribosomes in the present structure and with measurements on paused polysomes [18] . These considerations imply a direct mRNA transfer between consecutive ribosomes ( Fig. 3a ) in its unfolded state and exclude the possibility of a zigzag path of the mRNA between the ribosomes within the helix. The reason for this is that the continuous mRNA channel maintains the mRNA inside and prevents it from looping outside between ribosomes. As a result, within the polysome there is no need for helicase activity to unfold secondary mRNA structures [18] . An additional aspect is that forming a continuous channel probably helps protecting the mRNA from degradation. 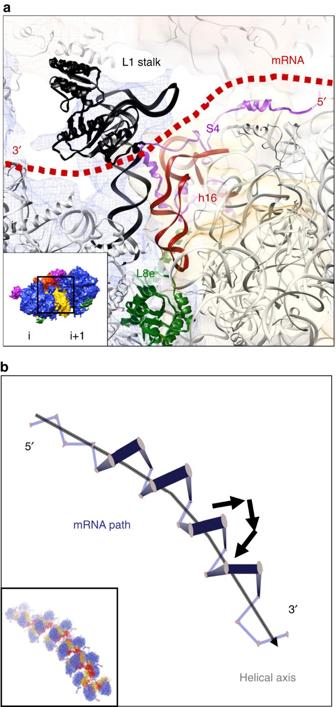Figure 3: Helical mRNA path through consecutive ribosomes. (a) Region of mRNA exit at the ribosomal platform and mRNA entry at the following (i+1) ribosome, revealing a direct transfer between consecutive ribosomes, which prevents the mRNA from looping between ribosomes (the putative mRNA path is indicated by a thick-dotted line in red, going from the downstream leading (i) ribosome to the subsequent upstream (i+1) ribosome from the 3′ end to the 5′ direction). (b) The overall mRNA path in the polysome as inferred from the relative positions of the ribosomes (the reference point is the decoding site in each ribosome). Because the ribosomes form a quasi-continuous channel for the mRNA, the mRNA path becomes twisted and follows the helical symmetry of the polysome (shown as insert). Arrows indicate the consecutive ribosomes in direction of their movement towards the mRNA 3′-termination region. Figure 3: Helical mRNA path through consecutive ribosomes. ( a ) Region of mRNA exit at the ribosomal platform and mRNA entry at the following (i+1) ribosome, revealing a direct transfer between consecutive ribosomes, which prevents the mRNA from looping between ribosomes (the putative mRNA path is indicated by a thick-dotted line in red, going from the downstream leading (i) ribosome to the subsequent upstream (i+1) ribosome from the 3′ end to the 5′ direction). ( b ) The overall mRNA path in the polysome as inferred from the relative positions of the ribosomes (the reference point is the decoding site in each ribosome). Because the ribosomes form a quasi-continuous channel for the mRNA, the mRNA path becomes twisted and follows the helical symmetry of the polysome (shown as insert). Arrows indicate the consecutive ribosomes in direction of their movement towards the mRNA 3′-termination region. Full size image The present work reveals one major ribosome conformation within the regular organization of the polysome, consistent with a single functional state due to the presence of the antibiotic cycloheximide. A unique structural state could also arise from a synchronized slow down of the elongation rate when polyribosomes form helical arrays in which tightly packed ribosomes could interfere with each other. The process could be triggered by transient stalling of downstream ribosomes or by decelerating the termination process, which may be a plausible mechanism for translation regulation with the preservation of ready-to-start ribosomes. Indeed, the formation of helical polysomes goes along with the cessation of viral mRNA translation in infected cells [6] , or with a change of embryogenesis phase in cotton [19] and results in a slow down of the translation rate in a cell-free system ( Fig. 4 and ref. 20 ). The fact that helical arrangements have also been observed in human cells [9] highlights the functional relevance of the cell-free system used here. The functional implications of higher-order polysomes in the cellular context could be that they serve as paused complexes from which translation can start quickly again when required, allowing rapid, local activation of protein synthesis. An example of this idea was described in a recent publication [21] , suggesting that neurons translate synaptic mRNAs upon synaptic signalling using stalled polyribosomes to bypass the rate-limiting step of translation initiation. Finally, the formation of a continuous mRNA channel system could have important functional implications in that it could serve to protect the mRNA from degradation. This concept appears particularly relevant for polysomes that serve as paused mRNA complexes in which the mRNA needs to remain protected until translation starts again. Related with this is the observation that the tight ribosome packing and the above considerations of the average inter-ribosome mRNA base-pair length located inside the channel would not allow the mRNA to loop outside the polysome assembly. This is consistent with the idea of mRNA protection, and in addition implies that no large secondary mRNA structures can form and thus there is no need for helicase activity and unfolding downstream mRNA secondary structures once the mRNA becomes polysome bound. The interplay between translation regulation and polysome structure will be an interesting aspect to analyze in future studies. 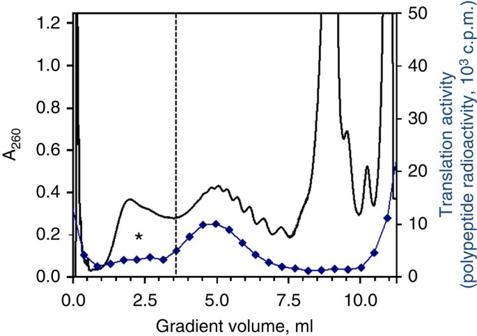Figure 4: Analysis of translation activity of different polysome fractions. The polyribosomes were formed during 2 h of 5′-UTRTMV-Luc-3′UTRTMVmRNA translation in the CECF format; then the reaction was transferred to batch format and, upon addition of [14C]amino acids (Ser+Phe), further incubation was followed for 8 min (one round of translation). Incorporation of TCA-precipitable radioactivity in the polypeptides synthesized by preformed polysomes was analyzed in gradient fractions after sedimentation of the reaction mixture in 15–50% sucrose gradient. The peak of fast sedimenting ‘heavy’ polysomes on the left of the dotted line (highlighted by the star) contains the densely packed heavy loaded polysomes. Figure 4: Analysis of translation activity of different polysome fractions. The polyribosomes were formed during 2 h of 5′-UTR TMV -Luc-3′UTR TMV mRNA translation in the CECF format; then the reaction was transferred to batch format and, upon addition of [14C]amino acids (Ser+Phe), further incubation was followed for 8 min (one round of translation). Incorporation of TCA-precipitable radioactivity in the polypeptides synthesized by preformed polysomes was analyzed in gradient fractions after sedimentation of the reaction mixture in 15–50% sucrose gradient. The peak of fast sedimenting ‘heavy’ polysomes on the left of the dotted line (highlighted by the star) contains the densely packed heavy loaded polysomes. Full size image Preparation of mRNA mRNA was prepared with the use of pTZβG-SBP-CBP-green fluorescent protein–N180 (GFP–N180) plasmid, containing under the control of the T7 promoter the following sequences: 5′ leader sequence of β-globin mRNA (rabbit), coding sequence of GFP (from pBAD–GFP vector, Maxigen) fused with the N-end SBP-CBP tag (from pCTAP-A vector, Stratagene) and C-terminal His6-tag. The plasmid was obtained from pTZβG-SBP-CBP–GFP–A30 plasmid (prepared on the basis of pTZ19R (Novagen) as described [22] by deleting the sequence between Bgl II and Xba I sites). In this way the A30 tail in the mRNA construct was removed and the non-specific 3′ untranslated region (UTR) could be generated from the plasmid sequence. The capped mRNA coding for N-tagged GFP (cap-5′UTR β-globin -scGFP–3′UTR N180, 1223 nucleotide (nt) total length, 975 nt of coding sequence) was prepared by in vitro transcription of pTZβG-SBP-CBP–GFP–N180 plasmid linearized at the Pvu I site, in the presence of 3′-O-Me-m 7 G(5′)ppp(5′)G cap-analogue. mRNA translation in the wheat germ cell-free system Wheat ( Triticum aestivum ) germ extract (220 OU 260 ml −1 ) was prepared and translation reactions were performed in continuous exchange cell-free (CECF) system according to the protocols described [23] . Briefly, the translation mixture contained 30% (v/v) wheat germ extract, 500 U ml −1 SUPERasin RNase inhibitor (Ambion), 100 μg ml −1 creatine phosphokinase, 50 μg ml −1 yeast total transfer RNA, 0.2 mM each 20 amino acids, 1 mM ATP, 0.4 mM GTP, 16 mM creatine phosphate and 25 mM HEPES-KOH buffer pH 7.6 with 3 mM Mg(OAc) 2 , 85 mM KOAc, 3 mM NaN 3 , 1.6 mM DTT, 0.25 mM spermidine and 2% glycerol. The reaction mixture was pre-incubated for 2 min at 25 °C before initiating the reaction at 25 °C by the addition of mRNA (final concentration 120 nM). The GFP synthesis was monitored by fluorescence measurement. Negative-staining EM The translation mixture with the polysomes was characterized by ultracentrifugation and negative-staining EM for initial visual quality control. For this, aliquots of translation mixture were diluted to 1.5 OU ml −1 with buffer A (25 mM HEPES-KOH pH 7.6, 5 mM Mg(Ac) 2 , 100 mM KAc, 0.03% NaN 3 and 0.01 mg ml −1 cycloheximide). The diluted samples (3 μl) were deposited on home-made grids with a thin layer of continuous carbon. After 1 min incubation the grid was blotted and 5 μl 2% uranyl-acetate was added. After 1 min, excess of the uranyl-acetate was blotted and the grid was dried. Observations of the sample were performed on the in-house CM120 or Tecnai F20 electron microscopes (Philips, Eindhoven, Netherlands), showing that the polysomes of various lengths and shape had formed, including characteristic long polysomes with over 20 regularly packed ribosomes that were next analyzed in detail by cryo-ET and sub-tomogram averaging. Cryo-ET and sub-tomogram averaging Higher-order polysomes were analyzed by cryo-ET and sub-tomogram averaging. Aliquots of the translation mixture after 6 h of reaction were diluted fivefold with buffer A. Colloidal gold markers (10 nm protein-A conjugate, purchased from the Department of Cell Biology, Utrecht University, the Netherlands) were added to give a final distribution of 6–25 beads per CCD field. The sample (3 μl) was applied to 300 mesh holey carbon homemade or Quantifoil 2/2 grids, blotted with filter paper from both sides for half a second in the temperature- and humidity-controlled Vitrobot apparatus (FEI, Eindhoven, Netherlands, T =20 °C, humidity 95%) and vitrified in liquid ethane pre-cooled by liquid nitrogen (see field of polysomes viewed by cryo-EM, Supplementary Fig. S1 ). CETs were recorded on the in-house Polara F30 S-FEG instrument (FEI) operating at 150 or 300 kV acceleration voltage and at a nominal underfocus of Δ z =−3 to −10 μm. Data acquisition was carried out using either CCD Eagle or a direct electron detector CMOS (Falcon 1) 4,096 × 4,096 camera (FEI; Supplementary Fig. S2 ) and control software for automated image tracking and focusing (FEI). Single-axis tilt series were recorded between −70° and +70° (±66° for the CCD data) with a tilt angle increment of 1°−3° and with the cumulative electron dose not exceeding 80 ē Å −2 at 300 kV and 30 ē Å −2 at 150 kV. The images were aligned by tracking ice-embedded gold markers using the FEI software Inspect3D (FEI) or IMOD [24] . To obtain the highest-resolution data, images were collected on the CMOS (rather than CCD) camera at defocus values of −3 μm using an acceleration voltage of 150 kV. Tomograms were coarsened by 2 or 4 and processed using the eTomo subroutine from the IMOD software package [24] ; final refinements and 3D reconstructions were run with uncoarsened data ( × 31,000 on the CMOS camera resulted in a pixel size at the specimen level of 3.4 Å, which represents a significant over-sampling with a Nyquist frequency of 6.8 Å compared with the resolution of the final map, see below). Sub-tomograms of the individual ribosomes were selected manually in IMOD and IMAGIC-V, extracted (box size 128, 3.4 Å per voxel, ribosome: ~90 pixels in diameter) and subjected to iterative alignment and averaging using the ml_tomo subroutine of the Xmipp software package, which involves template-free maximum-likelihood-based 3D alignment [25] , without needing a template or external reference structure which could otherwise introduce a bias during particle selection and averaging. Positioning of the sub-tomogram average back into the tomogram was done with Chimera software [27] . To address whether structural differences between individual ribosomes exist, a 3D classification of the maximum-likelihood-based sub-tomogram averaging of single ribosomes was done; it provided essentially identical 3D class averages, suggesting that no major conformational differences occur between ribosomes; this is consistent with the presence of elongation-state paused ribosomes adopting a similar conformation, for example, with respect to relative orientations of the ribosomal subunits. The sub-tomogram averaging largely removed missing wedge effects because of the different particle orientations. To reduce distortions in the reconstruction we also used dual-tilt series data collection (a combination of two single-tilt series collected separately on the same area of the specimen with an in-plane specimen rotation of 90°), a technique which significantly improves the tomogram quality also for single particle reconstructions [26] . Dual-tilt tomograms were used for particle identification and orientation search for sub-tomogram averaging applied to the first tilt series. Dual-tilt data were collected on CCD camera with a defocus of −3 μm using an acceleration voltage of 150 kV and a magnification of 39,000 (3.1 Å pixel −1 ) with a cumulative electron dose not exceeding 60 ē Å −2 , with fine angular increments of 1.5° with maximum tilt angle of ±70° for the first tilt series, and 3° increments with ±60 maximum tilt for the second tilt series (larger angular sampling in the second tilt series was shown to be sufficient for improving the overall tomogram reconstruction and allows reducing the dose [26] ). In total, about 90 wheat germ polysomes were reconstructed from single-tilt (CMOS: 7 tomograms at 150 kV, 10 tomograms at 300 kV, CCD: 60 tomograms at 150 kV) and 8 dual-tilt tomograms (each tomogram contained several polysomes). Over 20 polysomes were analyzed by sub-tomogram averaging, and they showed the same pattern of inter-ribosome interactions; in addition, we calculated a sub-tomogram average using a larger box to accommodate 5–7 ribosomes (box size 64, coarsened to 14.8 Å per voxel for faster calculation, ribosome: ~20 pixels in diameter): the obtained sub-tomogram average shows two ribosomes on either side of the central ribosome with relative angles and positions corresponding to those observed in the polysome helix reconstructed from individual ribosome sub-tomogram averages (see Supplementary Fig. 4 ), suggesting one main helical conformation and a rather strong conservation of the helical organization within the rather closely packed helical array. Three slices through the sub-tomogram shown in Fig. 1 also highlight the main inter-ribosome contacts (see Supplementary Fig. 5 ). The resolution of the sub-tomogram was estimated to ~26 or 34 Å according to the 0.143 criteria and 0.5 by Fourier-shell correlation (FSC, see Supplementary Fig. 6 ) of sub-tomogram averages from two independent sets of ribosome particles in the tomograms (only 106 particles in total; the small particle number may weaken the low-frequency components of the FSC, which tends to lead to an underestimation of the resolution; as mentioned above, the usage of a small number of particles for sub-tomogram averaging was done on purpose to get a more detailed map from data, as consistent as possible, originating from a single tomogram). The Imagic-V software package [28] was used for handling maps (filtering and masking; dilated mask derived from the map itself), for file format conversions and for FSC calculations. The combination of cryo-ET, sub-tomogram averaging and molecular modelling used here extends the integrated structural biology approach we recently used for isolated bacterial and human ribosome complexes [29] , [30] towards molecular assemblies. Map interpretation The interpretation of the obtained 3D structures was done by fitting available X-ray and high-resolution cryo-EM structures of wheat germ and yeast ribosomes (PDB IDs 3U5B, C, D, E, F, G, H, I, 3O2Z, 3O5H, 3O30, 3O58 and 3IZ6, 3IZ7, 3IZ9) [13] , [14] into the individual ribosome densities of the polysome. The analysis of the mRNA path was done according to the appropriate orientation and the shortest distance of the adjacent ribosomes for connecting the mRNA chain according to the 30S subunit part of the fitted crystal structure of the 70S mRNA complex [31] (PDB code 2HGP). Distances were measured and figures were prepared using the software Chimera [27] . Accession codes: The tomogram map and the coordinates of the fitted atomic model have been deposited in the EM Data Bank under the accession number EMD-2790 and in the Protein Data Bank under the accession number 4V3P . How to cite this article: Myasnikov, A. G. et al. The molecular structure of the left-handed supra-molecular helix of eukaryotic polyribosomes. Nat. Commun. 5:5294 doi: 10.1038/ncomms6294 (2014).